Deep proteome profiling ofTrichoplax adhaerensreveals remarkable features at the origin of metazoan multicellularity Genome sequencing of arguably the simplest known animal, Trichoplax adhaerens , uncovered a rich array of transcription factor and signalling pathway genes. Although the existence of such genes allows speculation about the presence of complex regulatory events, it does not reveal the level of actual protein expression and functionalization through posttranslational modifications. Using high-resolution mass spectrometry, we here semi-quantify 6,516 predicted proteins, revealing evidence of horizontal gene transfer and the presence at the protein level of nodes important in animal signalling pathways. Moreover, our data demonstrate a remarkably high activity of tyrosine phosphorylation, in line with the hypothesized burst of tyrosine-regulated signalling at the instance of animal multicellularity. Together, this Trichoplax proteomics data set offers significant new insight into the mechanisms underlying the emergence of metazoan multicellularity and provides a resource for interested researchers. Recently, the genomes of several phyla located near the base of the metazoan phylogenetic tree have been sequenced, including Porifera , Ctenophora , Cnidaria and Placozoa [1] . The placozoan genome is by far the smallest of these and has been regarded as the best living surrogate for the hypothetical Cnidaria – Bilateria ancestor genome, or even metazoan genome in general [2] , [3] . The placozoan Trichoplax adhaerens is morphologically the simplest of all animals, lacking a body axis, basal lamina and extracellular matrix (ECM), and containing only five somatic cell types [4] . It can be found in tropical and subtropical sea waters, and appears as a flat disc of 2–3 mm diameter consisting of two epithelial layers with a loose layer of fibre cells in between [5] . Trichoplax reproduces in vitro by fission and budding, and although in vitro the egg stadium does not develop into an embryonic stage beyond 64–128 cells, there are clear indications for a bisexual reproduction cycle, which left its signature in the DNA [6] , [7] . The Trichoplax genome contains 11,500 genes and, interestingly, includes importants genes characteristic of more complex bilaterian animals, such as developmental signalling pathways, neuroendocrine processes and extracellular matrix proteins [1] . The available genome, however, does not reveal which proteins are expressed, to what level and whether proteins are functionally regulated by posttranslational modifications (PTMs). Using high-resolution mass–spectrometry (MS)-based proteomics, we monitor for the first time which of the Trichoplax genes are actually translated and expressed. Moreover, as the functionality of proteins is to a large extent determined by PTMs, which can only be studied at the protein level, we look into more detail at some important PTMs, such as phosphorylation and acetylation. In summary, here we show that studying the proteome of Trichoplax , one of the most ancient extant multicellular animals, may provide significant insight into the mechanisms underlying the emergence of metazoan multicellularity. Expression abundance of 6,500 Trichoplax proteins We initially used 2,800 hand-picked animals of Trichoplax adhaerens and combined two independent enzymatic digestions, using trypsin and Lys-N, with strong cation exchange (SCX) peptide fractionation, nano reversed-phase liquid chromatography and high-resolution MS (LC-MS) to confidently identify 6,516 proteins at a false-discovery rate (FDR) of less than 1% ( Supplementary Data 1 ). This first extensive catalogue of proteins expressed by Trichoplax constitutes 57% of all predicted proteins and reveals similar qualitative features as the published in-depth proteome of C. elegans ( Fig. 1 ). The high-quality data set allows determination of individual protein expression abundance as described previously [8] , which covers over four orders of magnitude ( Fig. 2 ). A confirmation of the expression abundance was obtained using a bioduplicate experiment, performed 6 months later using a new batch of 1,000 hand-picked animals ( Supplementary Fig. S1 ). 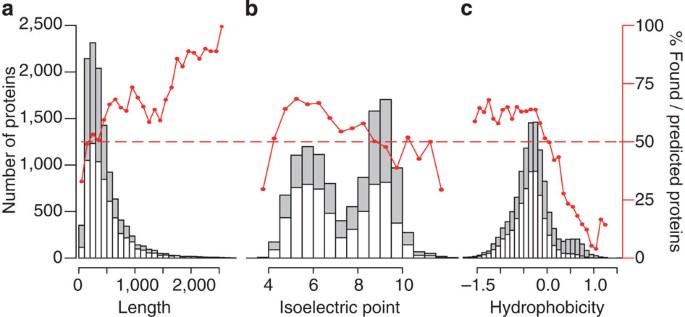Figure 1: Bias analysis of all identifiedTrichoplaxproteins. Properties for all proteins in SwissProt were calculated with BioPython 1.58 module ProtParam and plotted as a histogram (grey bars, corresponding to the left vertical axis). The analysis was repeated for all significantly detected proteins (white bars overlapping the grey bars). The proportion of the known and detected proteins for each histogram bar was calculated and depicted as red dots (rightmost axis), connected with lines for clarity. (a) There is a clear preference for detection of longer proteins by bottom-up mass spectrometry, which is in accordance with the notion that longer proteins yield more peptides, hence are more likely to be detected. (b) The isoelectric point does not have a clear influence on mass spectrometry coverage, which is around 50%. (c) A clear preference for hydrophilic proteins exists in our analysis. Figure 1: Bias analysis of all identified Trichoplax proteins. Properties for all proteins in SwissProt were calculated with BioPython 1.58 module ProtParam and plotted as a histogram (grey bars, corresponding to the left vertical axis). The analysis was repeated for all significantly detected proteins (white bars overlapping the grey bars). The proportion of the known and detected proteins for each histogram bar was calculated and depicted as red dots (rightmost axis), connected with lines for clarity. ( a ) There is a clear preference for detection of longer proteins by bottom-up mass spectrometry, which is in accordance with the notion that longer proteins yield more peptides, hence are more likely to be detected. ( b ) The isoelectric point does not have a clear influence on mass spectrometry coverage, which is around 50%. ( c ) A clear preference for hydrophilic proteins exists in our analysis. 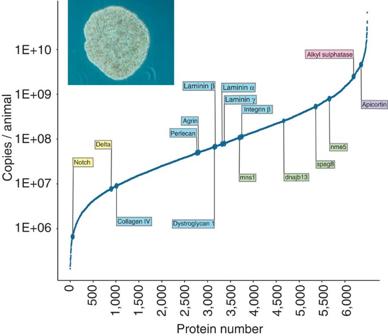Figure 2: An in-depth quantitative view of theTrichoplaxproteome. Protein copy numbers per animal of all identified proteins were estimated based on spectral counts as described in the Methods section. Selected proteins are highlighted and coloured by functional grouping as annotated in the KEGG31reference pathway maps: yellow for proteins belonging to the Notch signalling pathway, blue for ECM and adhesion-related proteins, green for male germ line markers, and pink and purple for alkyl sulphatase and apicortin. Inset photograph:Trichoplaxanimal in culture. Full size image Figure 2: An in-depth quantitative view of the Trichoplax proteome. Protein copy numbers per animal of all identified proteins were estimated based on spectral counts as described in the Methods section. Selected proteins are highlighted and coloured by functional grouping as annotated in the KEGG [31] reference pathway maps: yellow for proteins belonging to the Notch signalling pathway, blue for ECM and adhesion-related proteins, green for male germ line markers, and pink and purple for alkyl sulphatase and apicortin. Inset photograph: Trichoplax animal in culture. Full size image Observation of complex protein-mediated regulatory processes Detailed inspection of the expression abundance of Trichoplax proteins provides a wealth of information, strengthening evolutionary insights through the addition of an extra layer of information, including the occurrence of posttranslational events and confirmation of hypothesized gene expression. For instance, our data contain clear evidence for the abundant expression of ‘apicortin’, a unique protein with a putative cytoskeletal role shared only by apicomplexan parasites and Trichoplax [9] . And although there has been indirect evidence for a sexual life cycle in Trichoplax , five conserved sperm markers characteristic for different stages in spermatogenesis have only recently been identified [6] , four of which we can now confirm as being expressed abundantly at the protein level. Our data also provide evidence for the expression of proteins annotated by the KEGG database as part of signalling pathways important for animal development and patterning, including Delta and Notch proteins from the Notch pathway ( Fig. 3 ) and some downstream proteins from the Notch, Wnt and transforming growth factor-β pathways ( Fig. 3 and Supplementary Fig. S2 ). The placozoan genome encodes orthologues for many typical bilaterian ECM proteins. However, a peculiarity among the Metazoa is that an ECM of any kind, including a basal lamina, has eluded detection in adult Trichoplax , raising the possibility for expression of the ECM in other hitherto unknown developmental or life-cycle stages. In contrast, the proteomics data confirm the presence of proteins involved in ECM and ECM receptor interactions, including integrin-β, laminins, collagen IV, perlecan, agrin and dystroglycan, although there is a possibility that these proteins have alternative functions and/or organization. Recently, it was argued that a classical type cadherin in complex with two armadillo-type catenins is a key element in the origin of metazoan multicellularity [10] . Here we only found proof for expression of the flamingo-type cadherin and not of the suggested classical cadherin. The expression of the two armadillo-type catenins p120ctn and β-catenin could not be confirmed by our proteomics data. 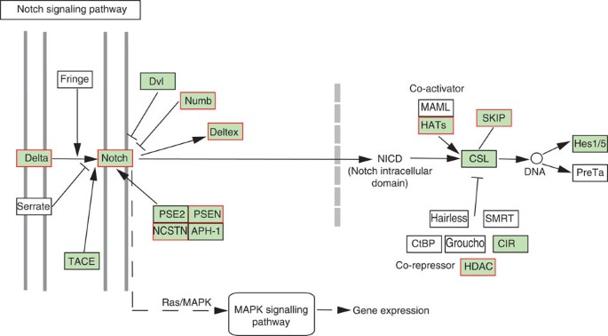Figure 3: The Notch signalling pathway map. Our protein identifications are mapped onto the KEGG31reference pathway maps athttp://www.genome.jp/kegg/kegg2.html. Colour green indicates the annotation of a Trichoplax orthologue in KEGG, red indicates identification of theTrichoplaxorthologue in our data set. Figure 3: The Notch signalling pathway map. Our protein identifications are mapped onto the KEGG [31] reference pathway maps at http://www.genome.jp/kegg/kegg2.html . Colour green indicates the annotation of a Trichoplax orthologue in KEGG, red indicates identification of the Trichoplax orthologue in our data set. Full size image Abundant presence of PTMs Although not specifically targeted, in-depth sequencing the Trichoplax proteome additionally allowed us to detect numerous protein PTMs, including widespread N-acetylation, lysine acetylation and phosphorylation. To focus on the latter, we detected, using an FDR<1% 2,177 unique phosphosites using SCX-based proteomics strategies. This number is similar to what we expect if an identical amount of mammalian sample is analysed using the same experimental approach [11] . At the same time, our quantitative proteomics data allowed us to define a semi-quantitative kinome tree for Trichoplax , depicted in Fig. 4b , in which detection and abundance in our proteome data set are shown for each kinase present in the Trichoplax genome ( Supplementary Data 2 ). Many Trichoplax kinases show high homology with human kinases ( Fig. 4a and Supplementary Fig. S3 ), and abundant kinases in our data set are orthologues to, for instance, protein kinase C, mitogen-activated protein kinase, CamK, AKT, CK2 and Src. Not surprisingly, motifs of abundant kinases, such as the CK2, mitogen-activated protein kinase and the Src family kinases were also abundantly recognized in the Trichoplax phosphopeptide data set. Strikingly, combining the data of three independent SCX phospho data sets ( Fig. 5 and Supplementary Data 3 ), serine accounted for 1,432 (66%) of the phosphosites, threonine for 555 (25%) and tyrosine for 190 (9%). The latter number of ~9% (respectively, 8.9%, 7.3% and 9.8% in the three independent SCX-based experiments) is extremely high and consisted of 166 unique proteins for which 95 human orthologues could be found, almost all of which (95%) have been reported to be phosphorylated on tyrosine residues as well ( Supplementary Data 4 ) [12] . Using similar experimental approaches, ~2% tyrosine phosphorylation is generally reported in dozens of phosphoproteomic studies on higher organisms ranging from C. elegans to humans [11] , [13] , [14] , [15] . 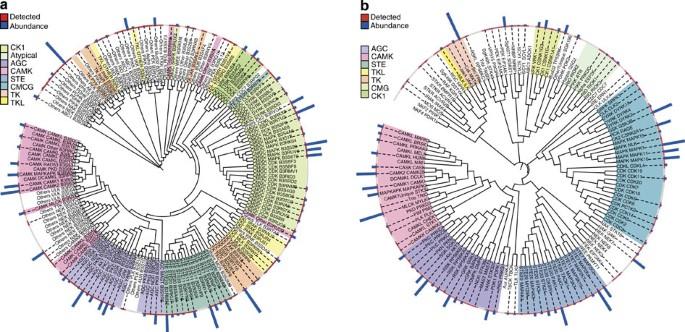Figure 4: A quantitative view of theTrichoplaxkinome. (a) Expression ofTrichoplaxkinases with Human orthologues. Human protein kinase orthologues for allTrichoplaxprotein kinases were determined by Inparanoid34. FASTA sequences of the kinase domains of the human orthologues were retrieved from the KinBase resource (http://kinase.com/kinbase/) and visualized as ina. Human orthologue names are listed by their grouping into kinase groups and families. (b) All identified kinases were ordered by phylogenetic distances of the kinase sequences. The FASTA sequences of all proteins designated by the KEGG31database as protein kinase (http://www.genome.jp/kegg-bin/get_htext?tad01001) were aligned using ClustalX2.1 (ref.32) using default parameters for multiple alignment and bootstrapping. For visualization, a phylogenetic tree was calculated with the neighbour-joining algorithm, exported and loaded into the Interactive Tree of Life tool33. Kinase families are coloured as defined by the KEGG31database. On the outer rim the colour red indicates that the kinase is detected, blue bars indicate the relative abundances in protein copy number per animal. Kinases are named according to their respective group, followed by family and finally their Uniprot accession number. Figure 4: A quantitative view of the Trichoplax kinome. ( a ) Expression of Trichoplax kinases with Human orthologues. Human protein kinase orthologues for all Trichoplax protein kinases were determined by Inparanoid [34] . FASTA sequences of the kinase domains of the human orthologues were retrieved from the KinBase resource ( http://kinase.com/kinbase/ ) and visualized as in a . Human orthologue names are listed by their grouping into kinase groups and families. ( b ) All identified kinases were ordered by phylogenetic distances of the kinase sequences. The FASTA sequences of all proteins designated by the KEGG [31] database as protein kinase ( http://www.genome.jp/kegg-bin/get_htext?tad01001 ) were aligned using ClustalX2.1 (ref. 32 ) using default parameters for multiple alignment and bootstrapping. For visualization, a phylogenetic tree was calculated with the neighbour-joining algorithm, exported and loaded into the Interactive Tree of Life tool [33] . Kinase families are coloured as defined by the KEGG [31] database. On the outer rim the colour red indicates that the kinase is detected, blue bars indicate the relative abundances in protein copy number per animal. Kinases are named according to their respective group, followed by family and finally their Uniprot accession number. 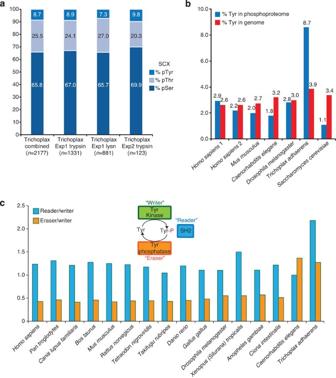Figure 5: A burst of tyrosine phosphorylation inTrichoplax. (a) Replicate measurements of tyrosine phosphorylation by SCX; in the first bar is the combined result of three independent SCX experiments (n=2177), in the second bar is the first trypsin experiment (n=1331), in the third bar is the Lys-N experiment (n=881) and in the fourth bar is an additional trypsin repeat experiment (n=123);n=total number of unique phosphosites (S, T, Y). (b) Compared with other organismsTrichoplaxexhibits a high percentage (3.9%) of tyrosine amino acids in its genome (red bars). The percentage of detected tyrosine phosphosites inTrichoplaxphosphoproteomics data sets is four- to fivefold higher than detected in large-scale phosphoproteomics data sets for other organisms, includingH. sapiens14,35,M. musculus13,D. melanogaster11andS. cerevisiae36(blue bars,Supplementary Data 4). Only species for which comprehensive protein phosphorylation data is also available, obtained using alike protocols, are shown37,38,39,40,41. (c)Trichoplaxcontains a relative high number of readers (SH2 phosphotyrosine recognition domains) and erasers (tyrosine phosphatases), compared with writers (tyrosine kinases) involved in tyrosine signalling. Tyrosine-kinase domains, SH2 domains and protein tyrosine phosphatase domains were detected using HMM models from SMART28using the online SMART tool (http://smart.embl-heidelberg.de/). Inset shows phosphotyrosine signalling as a tripartite system comprising tyrosine kinase (writer), tyrosine phosphatase (eraser) and SH2 domain (reader). Full size image Figure 5: A burst of tyrosine phosphorylation in Trichoplax . ( a ) Replicate measurements of tyrosine phosphorylation by SCX; in the first bar is the combined result of three independent SCX experiments ( n =2177), in the second bar is the first trypsin experiment ( n =1331), in the third bar is the Lys-N experiment ( n =881) and in the fourth bar is an additional trypsin repeat experiment ( n =123); n =total number of unique phosphosites (S, T, Y). ( b ) Compared with other organisms Trichoplax exhibits a high percentage (3.9%) of tyrosine amino acids in its genome (red bars). The percentage of detected tyrosine phosphosites in Trichoplax phosphoproteomics data sets is four- to fivefold higher than detected in large-scale phosphoproteomics data sets for other organisms, including H. sapiens [14] , [35] , M. musculus [13] , D. melanogaster [11] and S. cerevisiae [36] (blue bars, Supplementary Data 4 ). Only species for which comprehensive protein phosphorylation data is also available, obtained using alike protocols, are shown [37] , [38] , [39] , [40] , [41] . ( c ) Trichoplax contains a relative high number of readers (SH2 phosphotyrosine recognition domains) and erasers (tyrosine phosphatases), compared with writers (tyrosine kinases) involved in tyrosine signalling. Tyrosine-kinase domains, SH2 domains and protein tyrosine phosphatase domains were detected using HMM models from SMART [28] using the online SMART tool ( http://smart.embl-heidelberg.de/ ). Inset shows phosphotyrosine signalling as a tripartite system comprising tyrosine kinase (writer), tyrosine phosphatase (eraser) and SH2 domain (reader). Full size image The study of such a simple and probably most ancient extant multicellular animal as Trichoplax is highly significant to gain insight into the emergence of metazoan multicellularity, early animal evolution and subsequent metazoan diversity. In addition, it can be used as a simple multicellular model system to shed light on the origins and functioning of many biological processes essential in higher metazoa, like cellular differentiation, cell–cell communication, development and basic animal patterning. Therefore, it was particularly interesting to observe expression of proteins important in processes thought to be characteristic of more complex bilaterian animals, such as genes involved in developmental signalling pathways, that is, Notch, Wnt and transforming growth factor-β pathways ( Fig. 3 and Supplementary Fig. S2 ). Also, although nerve cells and ECM seemed to be absent in Trichoplax , proteins involved with neuroendocrine processes as well as putative ECM proteins and other ECM components were observed. Ranking of all proteins based on the number of spectral counts, we detected a protein that is homologous to the Saccharomyces cerevisiae BDS1 alkyl sulphatase among the top ten proteins in all SCX experiments ( Supplementary Data 1 , Fig. 2 and Supplementary Fig. S1 ). Interestingly, this yeast protein has been identified as being acquired by horizontal gene transfer from proteobacteria [16] . The very abundant Trichoplax BDS1 enzyme belongs to a group of less well-characterized alkyl sulphatases known from yeast, bacteria and very few higher animals (for example, Pea aphid and Vase tunicate ) that feed on chloroplast-rich diets [17] . We hypothesize that the presence of this enzyme in Trichoplax is linked to its unique feeding mode and its food source. It has been suggested that the first animals that appeared were “grazers” feeding on the cyanobacterial and algal mats of the oceans [18] . In this context, Trichoplax has been associated with fossils of Dickinsonia , whose motile feeding mode most closely resembled that of Trichoplax [19] . It moves over and on top of its food, which is then digested externally by uptake of the released nutrients. Trichoplax still uses this very ancient feeding mode [20] . The food of the first animals consisted of phototrophic organisms containing chloroplasts, forming a source of sulpholipids and other long-chain alkyl sulphates [21] , [22] . The high abundance of the BDS1 enzyme, which is able to scavenge sulphate from organically bound sources, is an important advantage for an extremely primitive animal without a gut and its associated flora. Most unanticipated was the observation of the relatively high number of tyrosine phosphorylation sites (that is, ~9% of the observed phosphopeptides in the three individual SCX data sets, Fig. 5a ), especially when taking into account that no common tyrosine phosphorylation enrichment procedures [23] were used. To further independently confirm these high levels of tyrosine phosphorylation, we performed phosphopeptide enrichment experiments using Ti-IMAC affinity beads [14] . We performed these experiments, in duplo , on similar protein amounts of Trichoplax and human HeLa cell lysates. Although the sample amount was limited, we identified around 1,000 phosphopeptides in each of the four experiments ( Supplementary Fig. S4 and Supplementary Data 5 ). Using the Hela cells as a control revealed that the percentage of tyrosine-phosphorylated peptides, observed using Ti 4+ -IMAC, is reduced by twofold when compared with the SCX experiment (that is, from ~3 to 1.5% pTyr, see Supplementary Fig. S4 ). It is well known that by applying certain PTM-enrichment strategies one may introduce potential biases towards certain physicochemical properties of the targeted modification. In this specific case, our prior experience with Ti 4+ -IMAC elucidated that it favours serine and also threonine phosphorylation over tyrosine phosphorylation, as further evidenced here. Notwithstanding, the relative ratio of tyrosine-phosphorylated peptides detected in the Trichoplax Ti 4+ -IMAC phosphoproteomics experiments is still >twofold higher than detected in the human HeLa cell data sets, confirming independently that pTyr is relatively more present in Trichoplax . Why then does Trichoplax have such a high relative frequency of phosphorylation on tyrosine residues? Tyrosine phosphorylation provides a molecular system for transmitting cellular regulatory information that appeared ~600 million years ago, close to the appearance of Trichoplax , and has been associated with the advent of multicellularity [24] , [25] , [26] . The basic repertoire of metazoan tyrosine kinases already existed before the advent of metazoan multicellularity, before the divergence of filasterians from metazoa and choanoflagellates. However, at the onset of metazoan multicellularity, probably recruitment of receptor tyrosine kinases as a communication tool between cells led to huge diversifications of these kinases between pre-metazoan and metazoan lineages. [27] The current view is that tyrosine phosphatases and Src Homology 2 (SH2) domains had already evolved in earlier organisms before the appearance of dedicated protein tyrosine kinases. With that view in mind, we performed genome-wide analysis of the tyrosine content and the number of tyrosine kinases (‘writers’), SH2 domains (‘readers’) and phosphatase domain (‘erasers’) as predicted by SMART [28] , including genomes of 16 different species ( Fig. 5c and Supplementary Data 6 ). Of all species analysed, Trichoplax contains the highest percentage of tyrosine amino acids in the predicted proteins (that is, 3.9%), whereas these numbers drop to ~2.6% in mammals ( Fig. 5b ). As predicted by SMART, Trichoplax contains 11 tyrosine kinases, 24 SH2 domain containing proteins and 14 phosphatases. Most strikingly, the ratio of reader to writer is exceptionally high for Trichoplax ( Fig. 5c ), indicating that the substrate-to-enzyme ratio is very favourable, possibly forming the basis for the relatively high phosphotyrosine count in our data. Together, these data provide strong experimental support for the concept of a sudden burst in tyrosine phosphorylation signalling at the beginning of metazoan multicellularity, followed by a gradual streamlining of phosphotyrosine signalling after the appearance of tyrosine kinases by reducing the number of possible deleterious phosphorylation sites as tyrosine kinase numbers increase [24] , [25] , [26] , [29] . Our in-depth proteomics data also allow improvements to be made to the Trichoplax genome annotation and gene models by matching mass spectra directly onto the genome sequences ( Supplementary Fig. S5 ). Furthermore, besides the discussed highly remarkable features of the Trichoplax proteome, the presented data set also contains information on N-acetylation, lysine acetylation and the abundance of proteins involved in many different pathways, making the data set a resource for researchers interested in the mechanisms of the origin and diversification of metazoan multicellularity. Animal culture and collection Animals of the so-called ‘Grell’ [5] clone were cultured in artificial sea water (ASW) at 23 °C and at an light/day regime of 16:8 h. Animals were fed ad libitum on the green alga Pyrenomonas helgolandii , but starved for 24 h before protein extraction to avoid contamination with the food [5] , [6] . Approximately 2,800 individual animals grown at 200–300 animals/culture plate were transferred to sterile six-well plates and washed three times each on two successive days with sterile ASW. Afterwards, animals were transferred to a sterile 1.5-ml eppendorf tube (~400 animals per tube), pelleted using a table centrifuge and washed with cold ASW (4 °C). For the replicate experiment, approximately 1,000 animals were collected under the same conditions, delivering ~160 μg of protein. Sample preparation After the washing procedure, animal pellets were lysed in 8 M urea, 50 mM ammonium bicarbonate and EDTA-free protease inhibitor cocktail (Sigma). After homogenization, lysates were cleared by centrifugation at 13,000 g for 20 min at 4 °C and supernatant was snap-frozen until digestion. After reductive alkylation of cysteine residues using 2 mM dithiothreitol and 5 mM iodoacetamide, 180 μg protein from ~1,400 animals was digested with 2 μg Lys-C (Roche Diagnostics, Ingelheim, Germany) in 500 μl 8 M urea and 50 mM ammonium bicarbonate for 4 h at 37 °C, followed by digestion with 4 μg trypsin (Roche Diagnostics) in 2 M urea and 50 mM ammonium bicarbonate at 37 °C for 16 h. Consecutively, 225 μg protein was digested with 2.5 μg Lys-N (U-Protein Express, Utrecht, The Netherlands) in 8 M urea and 50 mM ammonium bicarbonate for 4 h at 37 °C, followed by digestion with 3.5 μg Lys-N for 16 h at 37 °C in 4 M urea and 50 mM ammonium bicarbonate. Peptides were desalted using 1 ml Sep Pack C18 columns (Waters), and separated by SCX using a Zorbax BioSCX-Series II column (0.8-mm inner diameter, 50 mm length, 3.5 μm). SCX solvent A consists 0.05% formic acid in 20% acetonitrile (ACN), whereas solvent B was 0.05% formic acid, 0.5 M NaCl in 20% ACN. The SCX salt gradient was as follows: 0–0.06 min (0–2% B); 0.06–10.06 min (2–3% B); 10.06–20.06 min (3–8% B); 20.06–30 min (8–20% B); 30–40 min (20–40% B); 40–46 min (40–90% B); 46–50 min (90% B). Fractionated peptides were dried and resuspended in 10% formic acid. Thirty-seven fractions from both digests were then each analysed twice by reversed-phase LC-MS/MS. Phosphopeptide enrichment Ti 4+ -IMAC material was prepared and used essentially as previously described by us [14] . Affinity material was loaded onto Gel-loader tip microcolumns using a C8 plug and ~1–2 cm length of material. The columns were pre-equilibrated with 2 × 30 μl of Ti-IMAC loading buffer (80% ACN, 6% trifluoroacetic acid (TFA)). Next, samples were resuspended in 60 μl loading buffer and loaded onto the equilibrated gel-loader tip microcolumns. Columns were sequentially washed with 60 μl of loading buffer, followed by washing with 60 μl of 50% ACN/0.5% TFA containing 200 mM NaCl, and additional washing by 60 μl of 50% ACN/0.1% TFA. The bound peptides were eluted by 20 μl of 5% ammonia, followed by a second elution with 80% ACN/6% TFA, into 20 μl of 10% formic acid and then stored at −20 °C for LC-MS analysis. Liquid chromatography–mass spectrometry Peptide fractions were analysed using an Agilent 1100-Series LC system coupled to an LTQ-Orbitrap mass spectrometer (Thermo Scientific, Bremen, Germany). The LC system was equipped with a 20 mm Aqua C18 (Phenomenex, Torrance, CA) trapping column (packed in-house, i.d., 50 μm; resin 5 μm) and a 400 mm ReproSil-Pur C18-AQ (Dr Maisch GmbH, Ammerbuch, Germany) analytical column (packed in-house, i.d. 50 μm; resin 3 μm). Trapping was performed at 5 μl min −1 for 10 min, and elution was achieved with a gradient of 0–13% B in 0.1 min, 13–28% B in 107 min, 28–50% B in 35 min and 50–100% B in 2 min. The flow rate was passively split from 0.35 ml min −1 to 50 nl min −1 . Nanospray was achieved using a coated fused silica emitter (New Objective, Cambridge, MA) (o.d., 360 μm; i.d., 20 μm, tip i.d. 10 μm) biased to 1.7 kV. The mass spectrometer was operated in data-dependent mode to switch between MS and MS/MS. The five most intense ions were selected for fragmentation in the linear ion trap using collisionally induced dissociation at a target value of 30,000. Database search and validation Spectra were processed with Maxquant software to generate peak lists, which were then analysed with Mascot search engine version 2.3.02 (Matrix Science, London, UK) using a concatenated forward/reverse database of the Trichoplax Triad1-best-proteins-fasta sequences, setting carbamidomethyl (C) as fixed, and oxidation (M) and acetylation (protein N-term) as variable modifications. Maximum two missed cleavages were allowed, peptide tolerance was set to 50 p.p.m. and MS/MS tolerance to 0.6 Da. For phosphorylation analysis, carbamidomethyl (C) was set as fixed, and phospho (STY) and oxidation (M) were set as variable modifications with maximum one missed cleavage allowed. For lysine acetylation analysis, carbamidomethyl (C) was set as fixed, and acetyl (K) and oxidation (M) were set as variable modifications with maximum two missed cleavages allowed. Search results were filtered with Rockerbox [30] to an FDR of 1% using the concatenated database decoy method. Protein abundance calculations Numbers of identified spectra were used to calculate protein abundances [8] . Briefly, abundance factors were calculated from the number of identified spectra of a particular protein, divided by its molecular weight, multiplied by 10 6 for clarity. The abundance factor of a particular protein as a fraction of the total sum of all abundance factors was multiplied by the total amount of protein material used in each experiment, and from this the protein copy numbers were calculated by dividing by the protein molecular weights. This was divided by the number of animals used to get the number of protein copies per animal. How to cite this article: Ringrose, J. H. et al . Deep proteome profiling of Trichoplax adhaerens reveals remarkable features at the origin of metazoan multicellularity. Nat. Commun. 4:1408 doi: 10.1038/ncomms2424 (2013).